Structure-guided development of heterodimer-selective GPCR ligands Crystal structures of G protein-coupled receptor (GPCR) ligand complexes allow a rational design of novel molecular probes and drugs. Here we report the structure-guided design, chemical synthesis and biological investigations of bivalent ligands for dopamine D 2 receptor/neurotensin NTS 1 receptor (D 2 R/NTS 1 R) heterodimers. The compounds of types 1–3 consist of three different D 2 R pharmacophores bound to an affinity-generating lipophilic appendage, a polyethylene glycol-based linker and the NTS 1 R agonist NT(8-13). The bivalent ligands show binding affinity in the picomolar range for cells coexpressing both GPCRs and unprecedented selectivity (up to three orders of magnitude), compared with cells that only express D 2 Rs. A functional switch is observed for the bivalent ligands 3b,c inhibiting cAMP formation in cells singly expressing D 2 Rs but stimulating cAMP accumulation in D 2 R/NTS 1 R-coexpressing cells. Moreover, the newly synthesized bivalent ligands show a strong, predominantly NTS 1 R-mediated β-arrestin-2 recruitment at the D 2 R/NTS 1 R-coexpressing cells. Gprotein-coupled receptors (GPCRs) form the largest family of membrane proteins [1] . Because of their diversity and critical involvement in numerous cellular signalling processes in both central nervous system (CNS) and periphery, GPCRs represent today’s most popular drug targets attracting interdisciplinary scientific attention. Consequently, large progress has been made in understanding GPCR structures and modes of function. A growing number of studies showed that GPCRs not only exist as isolated entities but also interact within the plasma membrane by forming receptor dimers or higher-order oligomers [2] , [3] , [4] , [5] . Besides enabling cross-talk between individual signalling networks, receptor dimerization can induce activation of alternative signalling pathways [6] , [7] , influence ligand pharmacology and is critical for receptor trafficking and function [3] . Dopamine D 2 receptors (D 2 Rs), which belong to the family A of GPCRs, regulate a large number of physiological functions and are involved in a number of neuropsychiatric disorders including schizophrenia and Parkinson’s disease. Along with numerous other GPCRs, D 2 Rs have been proven to form homodimers [8] , [9] and heterodimers [10] , [11] , [12] , [13] , [14] , and growing evidence indicates that altered D 2 R cooperativity may significantly contribute to CNS disorders [15] , [16] . Among receptors interacting with D 2 Rs in the CNS, the neurotensin receptor subtype 1 (NTS 1 R) together with its endogenous ligand, the tridecapeptide neurotensin, has gained substantial interest over the past decades. Both GPCRs are closely associated and highly co-localized in vivo [17] . For example, more than 80% of dopaminergic neurons in the mesolimbic system express NTS 1 R (ref. 18 ). Moreover, neurotensin was found to decrease the D 2 R-affinity for dopamine and other agonists in striatal [19] and co-transfected HEK 293 T membrane preparations [20] . Evidence for the physical intramembrane interaction of both receptors was also conferred by means of bioluminescence resonance energy transfer, co-immunoprecipitation and attenuation of dopaminergic signalling in co-transfected human cells [20] , [21] . Since central administration of the neuropeptide in animals can mimic the effects of neuroleptic treatment, neurotensin has been hypothesized to act as endogenous antipsychotic [22] . Powerful tools for studying GPCR dimerization are bivalent ligands consisting of two pharmacophores tethered by an appropriate linker [23] , [24] . Bivalent ligands bridging the proximate orthosteric-binding sites of a dimer provide valuable insights into the quaternary structure of receptor dimers and the functional relevance of GPCR dimerization. Because of their selective recognition properties, bivalent ligands can be used for a tissue-specific targeting of cells expressing an individual GPCR dimer. Pioneering work in this field was performed developing dimer-preferring ligands to investigate opioid receptor dimerization in vitro and in vivo [25] , [26] , [27] and further compounds were synthesized to target GPCR homo- and heterodimers [28] , [29] , [30] , [31] , [32] , [33] . In theory, bivalent ligands successfully bridging two binding sites of adjacent protomers should confer extremely high affinity (resulting from the total binding energy of two recognition elements) and thus selectivity for the heterodimer. Most of the previous reports have shown compounds with only modest preference for heterodimers over monomers. High-resolution crystal structures of GPCR-ligand complexes open new opportunities for the design of bivalent ligands. A carefully designed bivalent ligand bridging two neighboured receptor protomers should exhibit extremely high binding affinity. This approach should lead to high tissue selectivity between heterodimer-expressing cells and those that express only one individual receptor [6] . Our work presents heterobivalent D 2 R/NTS 1 R ligands of type 1-3 comprising NT(8-13), the active fragment of the neuropeptide neurotensin, covalently linked to three different D 2 R-specific pharmacophores. These newly synthesized bivalent compounds exhibit high selectivity up to three orders of magnitude and picomolar K i values in D 2 R/NTS 1 R-coexpressing cells compared with cells expressing D 2 R only. Using bivalent ligands containing an agonist D 2 R pharmacophore substructure, we demonstrate that G i /G o -promoted D 2 R signalling is attenuated in the D 2 R/NTS 1 R coexpressing cells, while the compounds behave as full dopamine receptor agonists in cells singly expressing D 2 R. Design To design heterobivalent ligands, we intended to connect three different D 2 R pharmacophores to the NTS 1 R agonist NT(8-13) via an affinity-generating biphenyltriazole-moiety (lipophilic appendage) [34] , [35] and ω-amino acid-functionalized polyethylene glycol (PEG) spacers ( Fig. 1 ). As D 2 R pharmacophores, we used the D 2 R/D 3 R antagonist eticlopride, co-crystallized in complex with D 3 R (ref. 36 ), the privileged structure of a phenylpiperazine-based scaffold [37] and an aminoindane-type agonist [32] . Suitable attachment points for the connection of the pharmacophores with the linker were identified using the crystal structures of NTS 1 R (refs 38 , 39 ) and D 3 R (ref. 36 ). Inspection of the crystal structures revealed that the N-terminus of NT(8-13) and the 4’-position of eticlopride are accessible from the extracellular side. In an effort to determine a suitable linker length, we generated a D 2 R/NTS 1 R heterodimer model ( Fig. 2 ) consisting of a D 2 R homology model [40] (which was based on the D 3 R crystal structure) and the NTS 1 R crystal structure [39] (Supplementary Note 1; Supplementary Tables 1,2; and Supplementary Fig. 1 ). As templates to build the dimer model, we considered 16 crystal structures of 12 different GPCRs displaying homodimers with 18 individual receptor orientations. We generated dimer models based on every template. Models were not considered further if they showed substantial clashes between the two receptors, as well as models revealing a high distance between the protomers or showing a low parallelism of the two protomers. Showing relatively high sequence similarity with D 2 R, the structure of a β 1 -adrenergic receptor (β 1 -AR) homodimer [41] was selected as a template for the generation of the heterodimer model. The crystal structure revealed a dimer interface involving transmembrane helix 1 (TM1), TM2 and helix 8 (H8) that was previously reported to be important for D 2 R dimerization [8] and validated by crosslinking studies at β1-AR (ref. 41 ). The model showed a minimum distance (beeline) of 42 Å between the attachment points of eticlopride and NT(8-13) ( Fig. 2 and Supplementary Note 2 ). However, docking of eticlopride with the affinity-generating biphenyltriazole-moiety into the heterodimer model revealed two reasons why a longer spacer length should be required. First, the binding pocket of D 2 R restricts the D 2 R-attachment in a position not facing straight towards NTS 1 R ( Supplementary Fig. 2a ) and in addition, the way is partially blocked by the extracellular loop 1 of D 2 R and the N-terminus of NTS 1 R, resulting in a total distance of ∼ 55 Å. We concluded that at least two PEG-units, in addition to the biphenyltriazole-based attachment, should be necessary to enable a bivalent-binding mode (ligand 1b ), while a ligand containing only one PEG-unit (ligand 1a , corresponding to a maximal linker length of ∼ 46 Å) should lack the ability to bridge the two binding sites and could thus serve as a control agent ( Supplementary Fig. 2b ). To determine an optimum linker length, we additionally designed compounds 1c and 1d bearing three and four units of the functionalized PEG-spacer, respectively. Using an identical approach, we designed the bivalent compounds of types 2 and 3 featuring phenylpiperazine- and aminoindane-based D 2 R pharmacophores. Here, the attachment points at the pharmacophores were identified based on docking studies ( Supplementary Note 2 and Supplementary Fig. 3 ). We performed molecular dynamics (MD) on the bivalent ligands 1b , 2b and 3b (400 ns for each compound) in complex with the generated heterodimer model, because flaws in the process of ligand design would potentially appear as instabilities in the simulation systems. All three systems adopted stable receptor–ligand complexes during this time (Supplementary Note 3; Supplementary Fig. 4; and Supplementary Data 1 , 2 , 3 ). 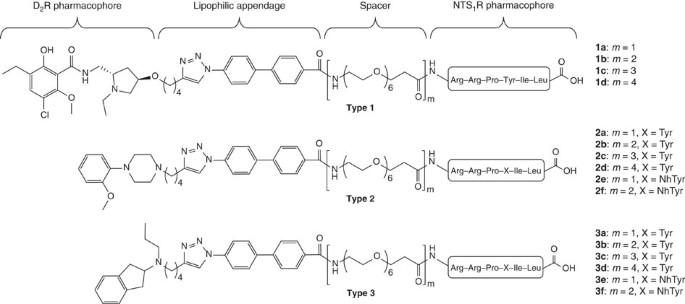Figure 1: Newly synthesized bivalent ligands. Type 1-3 ligands contain NT(8-13) as NTS1R pharmacophore and differ in their D2R recognition element (type 1: eticlopride, antagonist; type 2: 2-methoxyphenylpiperazine, antagonist; and type 3: aminoindane, agonist). The spacer length connecting both pharmacophores ranges from 22 to 88 atoms (m=1–4). For bivalent control compounds2e/fand3e/f, tyrosine was replaced by N-homotyrosine (NhTyr). Figure 1: Newly synthesized bivalent ligands. Type 1-3 ligands contain NT(8-13) as NTS 1 R pharmacophore and differ in their D 2 R recognition element (type 1: eticlopride, antagonist; type 2: 2-methoxyphenylpiperazine, antagonist; and type 3: aminoindane, agonist). The spacer length connecting both pharmacophores ranges from 22 to 88 atoms ( m =1–4). For bivalent control compounds 2e / f and 3e / f , tyrosine was replaced by N-homotyrosine (NhTyr). 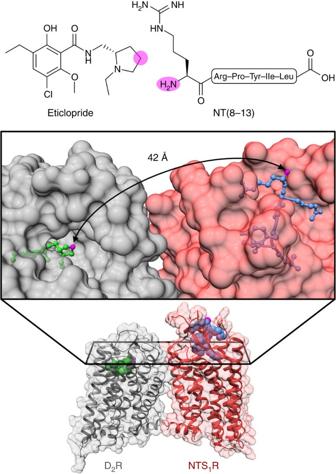Figure 2: A structure-guided approach for the design of bivalent ligands. On the basis of X-ray crystal structures, a D2R/NTS1R heterodimer model was generated and exploited for the design of bivalent ligands. A side view of dimer model is displayed at the bottom half and the ligand structures at the top of the figure. The middle part shows a magnified top view of the dimer model. Ribbons and surfaces of D2R and NTS1R are coloured in grey and red, respectively. Eticlopride (green) and NT(8-13) (blue) were positioned according to their coordinates in the crystal structures of D3R and NTS1R, respectively. Clearly, the N-terminus of NT(8-13) and the 4’-position of eticlopride are accessible from the extracellular side and were therefore selected as attachment points (highlighted as pink spots in all three representations). The beeline and hence the minimum distance connecting these two attachment points measures 42 Å. Full size image Figure 2: A structure-guided approach for the design of bivalent ligands. On the basis of X-ray crystal structures, a D 2 R/NTS 1 R heterodimer model was generated and exploited for the design of bivalent ligands. A side view of dimer model is displayed at the bottom half and the ligand structures at the top of the figure. The middle part shows a magnified top view of the dimer model. Ribbons and surfaces of D 2 R and NTS 1 R are coloured in grey and red, respectively. Eticlopride (green) and NT(8-13) (blue) were positioned according to their coordinates in the crystal structures of D 3 R and NTS 1 R, respectively. Clearly, the N-terminus of NT(8-13) and the 4’-position of eticlopride are accessible from the extracellular side and were therefore selected as attachment points (highlighted as pink spots in all three representations). The beeline and hence the minimum distance connecting these two attachment points measures 42 Å. Full size image Synthesis Chemical synthesis was conducted on solid phase involving the generation of the peptidic sequence, followed by ligation of the individual linker and coupling with the carboxylate-functionalized dopaminergic pharmacophore. The affinity-generating biphenyltriazole-moieties were installed using click chemistry. To generate appropriate control agents, we linked the dopaminergic building blocks to a peptide–peptoid hybrid of NT(8-13) (ref. 42 ), which is highly similar to NT(8-13) but shows only poor NTS 1 R affinity (compounds 2e , f , 3e , f ; Fig. 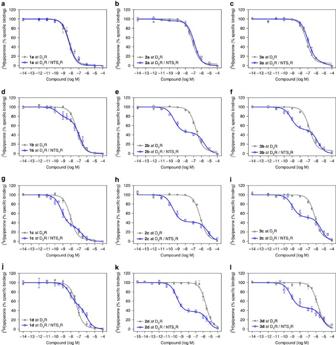Figure 3: Biphasic competition-binding curves indicate a bivalent binding mode. Dopamine receptor binding of the bivalent ligands1a–d,2a–dand3a–dwas measured by displacement of the radio-ligand [3H]spiperone from membranes of HEK 293 T cells coexpressing D2R/NTS1R (blue open circles) or monoexpressing D2R only (grey filled circles). (a-c) Bivalent ligands with a spacer length of 22 atoms (m=1) result in monophasic competition-binding curves. (d–l) Biphasic-binding curves indicating bivalent ligand binding are observed when the linker length is increased to 44, 66 or 88 atoms (m=2–4) at membranes coexpressing both target receptors (D2R/NTS1R) but not at membranes with D2R only. Data points represent the mean±s.e.m. of 3–22 independent experiments (seeTable 1for details), each performed in triplicate. 1 and Supplementary Table 3 ). Radio-ligand binding Binding profiles of the bivalent ligands of types 1–3 were determined by displacement of the radio-ligand [ 3 H]spiperone from the human D 2 R in membranes from HEK 293 T cells singly expressing the D 2 R and in D 2 R/NTS 1 R-coexpressing cells ( Table 1 ). Test compounds 1a , 2a and 3a containing biphenyltriazole-substituted eticlopride, phenylpiperazine and aminoindane moieties, respectively, linked to NT(8-13) by a short 22-atom spacer to NT(8-13) showed acceptable binding affinities to the D 2 R with K i values ranging from 1.4 and 1.7 nM for 1a up to double-digit nanomolar values for 2a and 3a , in D 2 R and D 2 R/NTS 1 R expressing membranes ( Table 1 and Fig. 3a–c ). Extension of the linker to 44 atoms resulted in comparable affinities for 1b , 2b and 3b at the D 2 R monoexpressing cells, ( K i 9.9, 42 and 36 nM). However, binding characteristics at the D 2 R/NTS 1 R-coexpressing cells were changed dramatically by the elongation of the linker. Thus, we observed biphasic competition curves with two individual values for K i high and K i low ( Fig. 3d–f ). For all three compounds, high-affinity binding was observed at subnanomolar concentrations ( K i high 0.11–0.47 nM) with a high-affinity population of 31–55%, while the affinity for the low-affinity site ranged from 43 to 630 nM ( Table 1 ). We suggest that the high-affinity K i values represent a bivalent receptor-bridging binding mode of 1b , 2b and 3b to D 2 R/NTS 1 R heterodimers, whereas low-affinity K i values reflect a monovalent-binding mode to D 2 R as a monomer or within a homo-/heterodimer. Thus, these newly designed ligands exhibit a 76–200-fold preference for the high-affinity bivalent interaction with the D 2 R/NTS 1 R heterodimer over monovalent-binding modes to D 2 R monoexpressing membranes. Table 1 D 2 R-affinity for ligands 1a–d, 2a–g and 3a–g determined by [ 3 H]spiperone displacement. Full size table Figure 3: Biphasic competition-binding curves indicate a bivalent binding mode. Dopamine receptor binding of the bivalent ligands 1a – d , 2a – d and 3a – d was measured by displacement of the radio-ligand [ 3 H]spiperone from membranes of HEK 293 T cells coexpressing D 2 R/NTS 1 R (blue open circles) or monoexpressing D 2 R only (grey filled circles). ( a - c ) Bivalent ligands with a spacer length of 22 atoms ( m =1) result in monophasic competition-binding curves. ( d – l ) Biphasic-binding curves indicating bivalent ligand binding are observed when the linker length is increased to 44, 66 or 88 atoms ( m =2–4) at membranes coexpressing both target receptors (D 2 R/NTS 1 R) but not at membranes with D 2 R only. Data points represent the mean±s.e.m. of 3–22 independent experiments (see Table 1 for details), each performed in triplicate. Full size image In contrast, the respective analogues 2e / f and 3e / f (spacer length 22 and 44 atoms), containing a peptide–peptoid hybrid with almost no affinity for NTS 1 R instead of the highly similar peptide NT(8-13), displayed monophasic-binding curves at both, D 2 R and D 2 R/NTS 1 R-coexpressing membranes ( K i 15-40 nM for D 2 R and K i 22–110 nM for D 2 R/NTS 1 R; Supplementary Fig. 5a–d ). Typical monophasic-binding curves were also observed for the monovalent analogues of types 2 and 3 ligands 2g and 3g for both expression systems ( K i 20 and 21 nM for 2g and 3g at D 2 R and K i 42 and 42 nM for 2g and 3g at D 2 R/NTS 1 R, respectively; Supplementary Fig. 5e,f ). In an attempt to find an optimum linker length, we also investigated the binding behaviour of compounds 1c – 3c and 1d – 3d with a spacer length of 66 and 88 atoms, respectively. Whereas ligands 1c and 1d maintained one-digit nanomolar affinity ( K i 2.5 and 9.0 nM), elongation of the spacer led to a loss of binding affinity for types 2 and 3 ligands ( K i 140–520 nM) at D 2 R monoexpressing membranes. Nevertheless, the biphasic-binding profiles with separated high- and low-affinity sites at D 2 R/NTS 1 R-coexpressing membranes were preserved or even enhanced for ligands 1c – 3c and 1d – 3d ( K i high 0.087–2.6 nM, K i low 120–1,800 nM, Fig. 3g–l ). Within the entire set of compounds, ligand 2d (spacer length 88 atoms) displayed the outstanding affinity of 87 pM for the high-affinity binding site. Interestingly, the preference for the high-affinity binding site versus the affinity for D 2 R monoexpressing membranes was more pronounced for types 2 and 3 ligands based on phenylpiperazines or aminoindane as D 2 R pharmacophores (76–4,700-fold), compared with the eticlopride-based derivatives (3.5–90-fold), with comparable fractions of high-affinity binding sites (50–66% high-affinity fraction). Additional binding assays were performed in the presence of an excess of NT(8-13) (1 μM), which should prevent a bivalent-binding mode of the test compounds to D 2 R/NTS 1 R-coexpressing membranes by displacing the NT(8-13) pharmacophore of the bivalent ligands from NTS 1 R. In fact, co-incubation prevented high-affinity binding, resulting in typical sigmoidal monophasic curves ( Fig. 4a and Supplementary Fig. 6a ). Detailed analyses revealed a slightly reduced D 2 R-affinity in the presence of the monovalent NTS 1 R agonist, which is in agreement with the reduced K i low observed for bivalent ligands at D 2 R/NTS 1 R-coexpressing membranes compared with D 2 R monoexpression ( Table 1 ). Importantly, these findings are consistent with earlier studies demonstrating a negative effect of neurotensin especially on D 2 R agonist affinity [19] , [20] . The binding properties of the reference antagonist spiperone remained almost constant under these conditions ( K i 0.073 and 0.080 nM, n =3, in the absence and presence of 1 μM NT(8-13), respectively). 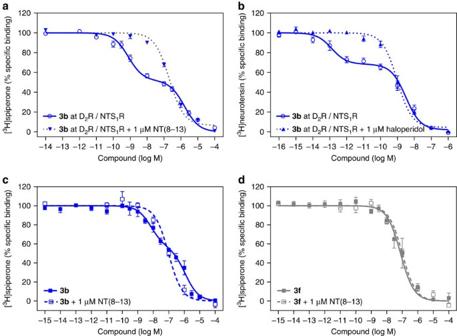Figure 4: Prevention of bivalent binding mode abolishes biphasic competition curves. (a) Dopamine receptor binding of3b(m=2, 44-atom spacer) at D2R/NTS1R in the absence (blue open circles) or presence (blue inverted triangles) of 1 μM NT(8-13). Incubation with the monovalent NTS1R agonist NT(8-13) prevents a bivalent binding mode and converts the biphasic-binding curve (Ki high0.47±0.14 nM,Ki low300±40 nM,n=22) into a monophasic sigmoid competition curve (Ki63±8 nM,n=6). (b) Neurotensin receptor binding of3b(m=2) at D2R/NTS1R in the absence (blue open circles) or presence (blue filled triangles) of 1 μM haloperidol. Incubation with the monovalent D2R antagonist prevents the bivalent binding mode, observed for the coexpression of D2R/NTS1R (Ki high0.11±0.05 pM,Ki low3.7±1.4 nM,n=9 versusKi0.79±0.21 nM,n=9). (c) When radio-ligand displacement studies were performed with striatal membranes and [3H]spiperone, biphasic-binding behaviour was observed for the bivalent ligand3b(blue filled squares,Ki high2.8±1.1 nM,Ki low310±90 nM, fraction high-affinity sites 38±5%,n=5) alone, but not in the presence of 1 μM NT(8-13) (blue open sqares,Ki28±3 nM,n=3). (d) For the bivalent control compound3fcomprising a peptoid-peptide hybrid instead of the NT(8-13) pharmacophore monophasic competition curves were observed in the absence (grey filled squares,Ki28±16 nM,n=5) and presence (grey open squares,Ki29±5 nM,n=4) of 1 μM NT(8-13). Data represent mean±s.e.m. ofnindependent experiments, each performed in triplicate. Figure 4: Prevention of bivalent binding mode abolishes biphasic competition curves. ( a ) Dopamine receptor binding of 3b ( m =2, 44-atom spacer) at D 2 R/NTS 1 R in the absence (blue open circles) or presence (blue inverted triangles) of 1 μM NT(8-13). Incubation with the monovalent NTS 1 R agonist NT(8-13) prevents a bivalent binding mode and converts the biphasic-binding curve ( K i high 0.47±0.14 nM, K i low 300±40 nM, n =22) into a monophasic sigmoid competition curve ( K i 63±8 nM, n =6). ( b ) Neurotensin receptor binding of 3b ( m =2) at D 2 R/NTS 1 R in the absence (blue open circles) or presence (blue filled triangles) of 1 μM haloperidol. Incubation with the monovalent D 2 R antagonist prevents the bivalent binding mode, observed for the coexpression of D 2 R/NTS 1 R ( K i high 0.11±0.05 pM, K i low 3.7±1.4 nM, n =9 versus K i 0.79±0.21 nM, n =9). ( c ) When radio-ligand displacement studies were performed with striatal membranes and [ 3 H]spiperone, biphasic-binding behaviour was observed for the bivalent ligand 3b (blue filled squares, K i high 2.8±1.1 nM, K i low 310±90 nM, fraction high-affinity sites 38±5%, n =5) alone, but not in the presence of 1 μM NT(8-13) (blue open sqares, K i 28±3 nM, n =3). ( d ) For the bivalent control compound 3f comprising a peptoid-peptide hybrid instead of the NT(8-13) pharmacophore monophasic competition curves were observed in the absence (grey filled squares, K i 28±16 nM, n =5) and presence (grey open squares, K i 29±5 nM, n =4) of 1 μM NT(8-13). Data represent mean±s.e.m. of n independent experiments, each performed in triplicate. Full size image However, even in the absence of NT(8-13), slight differences between the affinity for D 2 R monoexpressing membranes and the low-affinity binding site of D 2 R/NTS 1 R-coexpressing membranes were observed, suggesting that more complex ligand/receptor interactions might take place in the coexpressing membranes. Moreover, the simultaneous presence of at least three binding modes (bivalent and monovalent to D 2 R/NTS 1 R heterodimer, monovalent to D 2 R monomer) should putatively result in triphasic-binding curves, which we have not been able to resolve. Above described experiments were performed with a twofold excess of NTS 1 R, concluding that most of [ 3 H]spiperone-bound D 2 R were able to form D 2 R/NTS 1 R heterodimers. By changing the ratio towards a two- or three-fold excess of D 2 R, the high-affinity fraction, which corresponds to the bound receptor heterodimer, was rightward shifted and the biphasic character of the curve was gradually diminished ( Supplementary Fig. 6b ). Thus, a correlation between the ratio of protomers and the formation of molecular entities bound by bivalent ligands with particularly high affinity could be demonstrated. Further competition experiments with the bivalent ligands 2b and 3b were conducted in presence of the non-hydrolysable GTP analogue GppNHp, thereby destabilizing receptor-G protein association. In fact, co-incubation with 100 μM GppNHp had no influence on the binding behaviour of the bivalent ligand 2b at membranes from D 2 R-expressing cells ( K i – GppNHp 42±5 nM versus K i+GppNHp 45±6 nM). In contrast, a slight rightward shift of the K i was observed for compound 3b , which is in good agreement with its D 2 R agonist pharmacophore ( K i – GppNHp 36±9 nM versus K i+GppNHp 68±8 nM). However, at D 2 R/NTS 1 R-coexpressing membranes, a rightward shift of the high-affinity binding site occurred for both compounds (5.2- and 6.4-fold for 2b and 3b , respectively, Supplementary Fig. 7a,b ). These changes are expected, since the agonist NT(8-13) as NTS 1 R-recognizing fragment is part of both bivalent ligands, and agonist affinity is strongly dependent on the presence of G proteins. Nonetheless, in the presence of GppNHp, the biphasic-binding behaviour is retained, leading to a 330- and 190-fold preference for the high- over the low-affinity binding site in D 2 R/NTS 1 R-coexpressing membranes. To confirm the bivalent receptor-bridging binding mode, we performed reciprocal competition experiments by labelling the NTS 1 R with the radio-ligand [ 3 H]neurotensin. Therefore, we used a homogenate with a 2.5-fold excess of D 2 R. Employing 3b , we observed a biphasic-binding curve in cells expressing the D 2 R/NTS 1 R heterodimer with a K i high value of 0.11 pM and a K i low at 1.7 nM, which was shifted to a monophasic sigmoidal binding curve in the presence of haloperidol ( K i 0.79 nM, Fig. 4b ). Hence, incubation with the monovalent D 2 R antagonist efficiently prevented the bivalent-binding mode. Affinities for this competition-enforced monovalent-binding mode were found to be in good agreement with results obtained with membranes from CHO-cells stably expressing NTS 1 R only ( K i 0.86 nM; Supplementary Table 3 and Supplementary Methods ). To complement the results obtained with overexpressing heterologous cell lines with results from native brain tissue, competition-binding studies with [ 3 H]spiperone and the bivalent ligand 3b in comparison with the control agent 3f (both with a spacer length of 44 atoms) were performed with membranes from porcine striatum. Convincingly, test compound 3b displayed a biphasic-binding behaviour with a 140-fold preference for the high-affinity binding site over the low-affinity receptor population ( K i high 2.8 nM, K i low 310 nM, high-affinity fraction 38%). In good agreement with the results from heterologous cell lines, addition of 1 μM NT(8-13) reverted this biphasic-binding curve to a sigmoidal binding isotherm with a K i value of 28 nM. In contrast, typical monophasic-binding curves with K i values of 28 and 29 nM were observed in the absence and presence of 1 μM NT(8-13) for the highly similar peptide–peptoid hybrid ligand 3f , which proved to have almost no affinity for NTS 1 R ( Fig. 4c,d ). Thus, the connection of D 2 R- and NTS 1 R-addressing pharmacophores by an appropriate linker allows the superior recognition of heterodimers over monomers or homo(oligo-)mers not only in heterologous cell lines but also in native tissue. However, the observed preferences are less pronounced in striatal membranes, which might be, at least in part, explained by lower receptor expression levels leading to a lower propensity to form D 2 R/NTS 1 R heterodimers. Functional evaluation To measure activation profiles of the bivalent ligands 2b and 3b and their monovalent analogues 2g and 3g comprising the pharmacophore of a D 2 R antagonist and a D 2 R agonist, respectively, we performed a BRET-based cAMP accumulation assay [43] . Coupling to inhibitory Gα i/o proteins, the stimulation of the D 2 R leads to a decrease of cAMP, whereas activation of the Gα s -coupled NTS 1 R increases adenylyl cyclase activity. As expected, the reference agonist quinpirole potently inhibited forskolin-induced cAMP accumulation in cells expressing D 2 R only, while the phenylpiperazine-derived ligands 2b and 2g and the NTS 1 R-binding fragment NT(8-13) remained without significant effects ( Fig. 5a ). 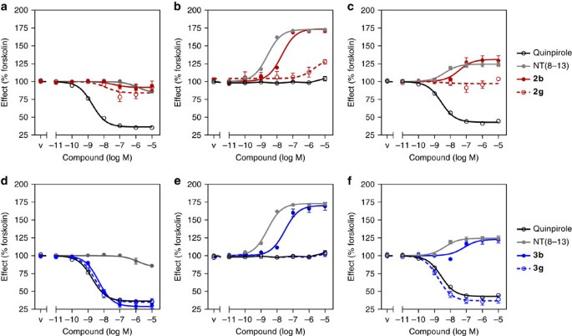Figure 5: Functional investigation (cAMP accumulation) for representative ligands. Functional activity of the bivalent ligands2b,3band their monovalent analogues2g,3gwas determined in HEK 293 T cells coexpressing the cAMP-BRET biosensor CAMYEL and the D2R (a,d), the NTS1R (b,e) or both D2R and NTS1R (c,f). Cells were stimulated with increasing amounts of the ligands in the presence of 10 μM forskolin. cAMP production was normalized to the percentage of forskolin-induced cAMP concentration (100%). (a) While quinpirole potently inhibited cAMP formation, both D2R antagonists2b,2gand the NTS1R agonist NT(8-13) remained without significant effect on cells expressing D2R. (b) NTS1R could be stimulated by NT(8-13) and the bivalent ligand2b, also bearing a NT(8-13) pharmacophore. (c) In the coexpressing cells, NT(8-13) induced an increase of cAMP, while quinpirole decreased the forskolin stimulated cAMP production. The bivalent ligand2balso increased the cAMP production, similar to cells expressing NTS1R only. (d) Ligands3band3ginhibited cAMP formation highly similar to quinpirole, revealing potent D2R agonism. (e) In cells monoexpressing NTS1R, only the bivalent ligand3bstimulated receptor activation, while the monovalent analogue3gcaused no effect. (f) While the monovalent ligand3gshowed an effect similar to quinpirole, the bivalent ligand3binduced further cAMP accumulation, indicating that its D2R-mediated effect was missing in the coexpressing cell line. Data represent mean±s.e.m. of 3–11 (for details seeSupplementary Table 4) independent experiments each performed in triplicate; v=vehicle (PBS+10 μM forskolin). Figure 5: Functional investigation (cAMP accumulation) for representative ligands. Functional activity of the bivalent ligands 2b , 3b and their monovalent analogues 2g , 3g was determined in HEK 293 T cells coexpressing the cAMP-BRET biosensor CAMYEL and the D 2 R ( a , d ), the NTS 1 R ( b , e ) or both D 2 R and NTS 1 R ( c , f ). Cells were stimulated with increasing amounts of the ligands in the presence of 10 μM forskolin. cAMP production was normalized to the percentage of forskolin-induced cAMP concentration (100%). ( a ) While quinpirole potently inhibited cAMP formation, both D 2 R antagonists 2b , 2g and the NTS 1 R agonist NT(8-13) remained without significant effect on cells expressing D 2 R. ( b ) NTS 1 R could be stimulated by NT(8-13) and the bivalent ligand 2b , also bearing a NT(8-13) pharmacophore. ( c ) In the coexpressing cells, NT(8-13) induced an increase of cAMP, while quinpirole decreased the forskolin stimulated cAMP production. The bivalent ligand 2b also increased the cAMP production, similar to cells expressing NTS 1 R only. ( d ) Ligands 3b and 3g inhibited cAMP formation highly similar to quinpirole, revealing potent D 2 R agonism. ( e ) In cells monoexpressing NTS 1 R, only the bivalent ligand 3b stimulated receptor activation, while the monovalent analogue 3g caused no effect. ( f ) While the monovalent ligand 3g showed an effect similar to quinpirole, the bivalent ligand 3b induced further cAMP accumulation, indicating that its D 2 R-mediated effect was missing in the coexpressing cell line. Data represent mean±s.e.m. of 3–11 (for details see Supplementary Table 4 ) independent experiments each performed in triplicate; v=vehicle (PBS+10 μM forskolin). Full size image Since we were unable to detect intrinsic activity for type 2 ligands in our cAMP accumulation assay, we tested the representative bivalent and monovalent ligands 2b and 2g for their capacity to prevent quinpirole-mediated inhibition of cAMP accumulation. As expected, both ligands were able to fully inhibit the effect of 10 nM quinpirole. In comparison, the type 1 ligand 1b and its pharmacologically active D 2 R fragment eticlopride were more potent and even showed an inverse agonist effect, leading to a 20–32% change in the basal cAMP level ( Supplementary Fig. 8 ). The bivalent ligand 3b and the monovalent dopaminergic 3g bearing the aminoindane moiety displayed functional properties that were highly similar to quinpirole. Observed potencies (EC 50 ) were in the low nanomolar range (2.3–5.0 nM), and maximum efficacies did not differ significantly among the three investigated D 2 R agonists ( Fig. 5d and Supplementary Table 4 ). In cells expressing only NTS 1 R, neither the monovalent ligands 2g , 3g , nor quinpirole were able to exhibit receptor activation. However, the bivalent ligands 2b and 3b were as effective as NT(8-13), albeit at 10-fold higher concentrations (EC 50 2.6 nM for NT(8-13) versus EC 50 20.7 and 30.6 nM for 2b and 3b, Fig. 5b,e ). In D 2 R/NTS 1 R-coexpressing cells, quinpirole and the monovalent D 2 R agonist 3g inhibited cAMP formation with similar potencies compared with cells monoexpressing D 2 R. The monovalent phenylpiperazine 2g had no effect on the intracellular cAMP concentration. Interestingly, all investigated bivalent ligands increased cytosolic cAMP in a similar manner as NT(8-13). Observed potencies were comparable to the monoexpressing NTS 1 R cells (EC 50 2.0 nM for NT(8-13) versus 39.3 and 70.0 nM for 2b and 3b , respectively), although a slight loss in potency could be observed for the bivalent ligands ( Fig. 5c,f ). The extremely high affinity of the bivalent ligands could not be transduced into an increase in potency at D 2 R/NTS 1 R-coexpressing cells. When the spacer connecting the D 2 R and NTS 1 R pharmacophores was elongated to 66 atoms for the bivalent ligands 2c and 3c , similar observations concerning the activation of D 2 R, NTS 1 R and D 2 R/NTS 1 R heterodimers were made ( Supplementary Fig. 9a–c and Supplementary Table 4 ). The absence of D 2 R-mediated inhibition of cAMP accumulation in cells coexpressing D 2 R/NTS 1 R, is not specific for bivalent ligands, since a comparable attenuation of dopaminergic signalling is achieved when D 2 R/NTS 1 R-coexpressing cells are stimulated with quinpirole and NT(8-13) simultaneously ( Supplementary Fig. 10a ). In contrast, a reciprocal inhibition of NTS 1 R signalling by increasing concentrations of D 2 R agonist could not be observed ( Supplementary Fig. 10b ). To exclude interference from forskolin stimulation or the relative receptor stoichiometry, experiments were also performed in the absence of forskolin and under conditions leading to enhanced NTS 1 R expression and therefore higher propensity to obtain D 2 R/NTS 1 R heterodimers. As illustrated in Supplementary Fig. 11a–e , these modifications did not result in significant changes of the receptor activation profiles of quinpirole, NT(8-13) or the bivalent ligands 2b and 3b . Coexpression of NTS 1 R and a signalling incompetent D 2 R-mutant (D80A) [44] , [45] led to a loss of dopamine receptor signalling for the monovalent dopaminergic 3g and quinpirole while preserving the above described biphasic-binding behaviour and the activation profile of bivalent ligand 3b ( Supplementary Fig. 12a,b ) in D 2 R_D80A/NTS 1 R-coexpressing cells. Besides G proteins, a class of adaptor proteins called β-arrestins are frequently found to interact with GPCRs. The recruitment of β-arrestin to a GPCR can lead to internalization but also initiate signalling events distinct from the G protein-mediated response [46] . To investigate the interaction of D 2 R/NTS 1 R heterodimers with β-arrestin-2, we made use of an assay system based on enzyme complementation (DiscoveRx PathHunter). Hence, HEK 293 cells stably expressing β-arrestin-2 fused to an enzyme acceptor (EA, galactosidase fragment) were transiently transfected with ProLink-tagged D 2 R together with or without cotransfection of wild-type NTS 1 R. Upon recruitment of β-arrestin-2 to D 2 R, the following enzyme complementation leads to conversion of a substrate and thereby chemiluminescence. The D 2 R agonist quinpirole induced β-arrestin-2 recruitment in D 2 R monoexpressing and D 2 R/NTS 1 R-coexpressing cells with similar potencies (EC 50 55±3 versus 75±11 nM). Interestingly, stimulation with NT(8-13) induced β-arrestin-2 recruitment in the coexpressing cells, but not cells singly expressing D 2 R, indicating that β-arrestin-2 recruitment by NTS 1 R can be detected if it occurs in close proximity of D 2 Rs, as for example within a D 2 R/NTS 1 R heterodimer. Although the maximum effect remained below the response of quinpirole (77±3%), NT(8-13) elicited that response at 10-fold lower concentrations (EC 50 7.5±2.1 nM; Fig. 6a,b ). Application of an equimolar combination of both agonists led to an even enhanced efficiency of β-arrestin-2 recruitment ( E max 136±6%; Supplementary Fig. 13a ). 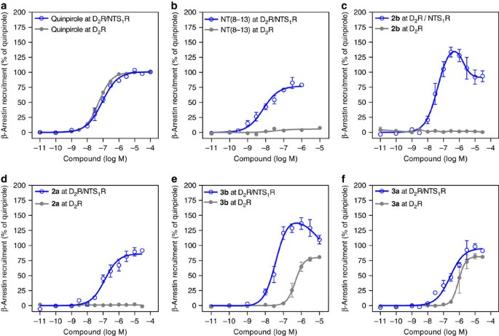Figure 6: β-Arrestin-2 recruitment at D2R and D2R/NTS1R heterodimers. β-Arrestin-2 recruitment was determined employing an assay based on enzyme complementation. HEK 293 cells stably expressing β-arrestin-2 tagged with the EA were transfected with ProLink-tagged D2R with (open blue circles) or without (filled grey circles) cotransfection of NTS1R (a) Quinpirole induces β-arrestin-2 recruitment in cells singly expressing D2R (n=9) and cells coexpressing D2R/NTS1R (n=11) with similar potencies. (b) NT(8-13) induces β-arrestin-2 recruitment with a maximum effect of 77±3% in cells coexpressing D2R/NTS1R (n=5), but not in D2R monoexpressing cells (n=4). (c) The phenylpiperazine-derived bivalent ligand2bhas no intrinsic activity in cells expressing D2R only (n=3), while it potently induces β-arrestin-2 recruitment in cells coexpressing D2R/NTS1R (n=7). Instead of a sigmoid curve, a bell-shaped dose–response profile is observed with a superior maximum effect as compared with both reference agonists. (d) The bivalent ligand2adoes not lead to β-arrestin-2 recruitment in D2R monoexpressing cells (n=3), but causes a typical sigmoid dose–response curve in the D2R/NTS1R-coexpressing cells (n=7). (e) The aminoindane-based bivalent ligand3binduces β-arrestin-2 recruitment in cells expressing D2R (n=4) and cells coexpressing D2R/NTS1R (n=6). Coexpression of NTS1R leads to a significant increase in potency and efficacy and a bell-shaped dose–response curve as observed inc. (f) The aminoindane-type agonist with a 22-atom spacer (3a) leads to β-arrestin-2 recruitment in both types of transfected cells (n=3 for D2R andn=5 for D2R/NTS1R). Data represent mean±s.e.m. ofnindependent experiments, each performed in duplicate. Results were normalized to the maximum effect of quinpirole (100% for D2R and D2R/NTS1R). Figure 6: β-Arrestin-2 recruitment at D 2 R and D 2 R/NTS 1 R heterodimers. β-Arrestin-2 recruitment was determined employing an assay based on enzyme complementation. HEK 293 cells stably expressing β-arrestin-2 tagged with the EA were transfected with ProLink-tagged D 2 R with (open blue circles) or without (filled grey circles) cotransfection of NTS 1 R ( a ) Quinpirole induces β-arrestin-2 recruitment in cells singly expressing D 2 R ( n =9) and cells coexpressing D 2 R/NTS 1 R ( n =11) with similar potencies. ( b ) NT(8-13) induces β-arrestin-2 recruitment with a maximum effect of 77±3% in cells coexpressing D 2 R/NTS 1 R ( n =5), but not in D 2 R monoexpressing cells ( n =4). ( c ) The phenylpiperazine-derived bivalent ligand 2b has no intrinsic activity in cells expressing D 2 R only ( n =3), while it potently induces β-arrestin-2 recruitment in cells coexpressing D 2 R/NTS 1 R ( n =7). Instead of a sigmoid curve, a bell-shaped dose–response profile is observed with a superior maximum effect as compared with both reference agonists. ( d ) The bivalent ligand 2a does not lead to β-arrestin-2 recruitment in D 2 R monoexpressing cells ( n =3), but causes a typical sigmoid dose–response curve in the D 2 R/NTS 1 R-coexpressing cells ( n =7). ( e ) The aminoindane-based bivalent ligand 3b induces β-arrestin-2 recruitment in cells expressing D 2 R ( n =4) and cells coexpressing D 2 R/NTS 1 R ( n =6). Coexpression of NTS 1 R leads to a significant increase in potency and efficacy and a bell-shaped dose–response curve as observed in c . ( f ) The aminoindane-type agonist with a 22-atom spacer ( 3a ) leads to β-arrestin-2 recruitment in both types of transfected cells ( n =3 for D 2 R and n =5 for D 2 R/NTS 1 R). Data represent mean±s.e.m. of n independent experiments, each performed in duplicate. Results were normalized to the maximum effect of quinpirole (100% for D 2 R and D 2 R/NTS 1 R). Full size image For the bivalent ligands of the phenylpiperazine-type 2a and 2b with 22- and 44-atom spacers, no β-arrestin-2 recruitment was observed in cells expressing D 2 R only, which is in good agreement with the antagonist properties observed for 2a and 2b in the cAMP accumulation assay. Interestingly, a bell-shaped dose–response curve was observed for the bivalent ligand 2b in D 2 R/NTS 1 R-coexpressing cells. Maximum β-arrestin-2 recruitment was determined at a concentration of 300 nM ( E max 133%), while higher ligand concentrations led to an attenuated response ( Fig. 6c ). In contrast, a typical sigmoid dose–response curve was observed for the analogue 2a with the shorter 22-atom spacer (EC 50 110±20 nM, E max 88±4%, Fig. 6d ). As expected, the bivalent ligands 3a and 3b bearing the aminoindane-type D 2 R agonist substructure elicited β-arrestin-2 recruitment in cells monoexpressing D 2 R (EC 50 1,500±500 nM, E max 87±5% and EC 50 580±130 nM, E max 82±1% for 3a and 3b respectively, Fig. 6e,f ). Highly similar to the activation profiles of type 2 compounds, a bell-shaped dose–response curve with a maximum effect at a concentration of 300 nM to 1 μM ( E max 136%) was observed when NTS 1 R was coexpressed for 3b (44-atom spacer), but not 3a (22-atom spacer, EC 50 37±8 nM, E max 105±9%, Fig. 6e,f ). Bell-shaped dose–response curves with enhanced efficacy were also observed for the bivalent ligands 2c and 3c (66-atom spacer; Supplementary Fig. 13b,c ). Additional experiments were performed employing a ProLink-tagged signalling incompetent D 2 R_D80A mutant coexpressed with NTS 1 R. Under these conditions, only NTS 1 R-mediated β-arrestin-2 recruitment can be detected. As expected, the NTS 1 R agonist NT(8-13), but not the D 2 R agonist quinpirole, was able to induce β-arrestin-2 recruitment in D 2 R_D80A/NTS 1 R-coexpressing cells. The potency of NT(8-13) was highly comparable to cells coexpressing wild-type D 2 R/NTS 1 R (EC 50 5.9±1.2 nM for D 2 R_D80A/NTS 1 R and EC 50 7.5±2.1 nM for wild-type D 2 R/NTS 1 R; Supplementary Fig. 14a,b ). Highly similar to the results obtained with intact D 2 R, bivalent ligands with a short spacer (22-atoms, 2a , 3a ) resulted in sigmoid dose–response curves (EC 50 67±23 nM, E max 98±4% and EC 50 190±40 nM, E max 113±7%, for 2a and 3a ) in cells coexpressing NTS 1 R with the signalling incompetent D 2 R mutant, while bell-shaped curves with increased maximum efficacy were observed for the ligands with the longer spacer ( 2b , c , 3b , c , 44- and 66-atom spacer, Supplementary Fig. 14c–h ). Ligands 2b , c and 3b , c reached maximum effects up to 210% relative to NT(8-13). When the same experiments were performed in HEK 293 cells coexpressing NTS 1 R with ProLink-tagged protease-activated receptor subtype 2 (PAR 2 ), only a very weak recruitment of β-arrestin-2 was observed for NT(8-13) and the representative bivalent ligands 2c and 3b (≤ 19%) compared with the PAR 2 agonist f-LIGRLO-NH 2 (ref. 47 ). The D 2 R agonist quinpirole was entirely inactive. Importantly, all dose–response curves showed a typical sigmoid profile ( Supplementary Fig. 15a–d ). These results indicate a specific effect of the bivalent ligands leading to bell-shaped dose–response curves in D 2 R/NTS 1 R-coexpressing cells. GPCR exist as monomers or cross-react forming dimers and higher-order oligomers. Because dimerization of GPCRs can result in modified ligand-binding and -signalling properties, a selective targeting of these entities is a powerful strategy in chemical biology and drug discovery. Irrespective of whether or not dimerization has physiological consequences per se , medicinal chemistry can take advantage of this phenomenon targeting drugs towards cells coexpressing an individual dimer-forming combination of GPCRs. In theory, bivalent ligands successfully bridging two binding sites of adjacent protomers should confer extremely high affinity (resulting from the total binding energy of two recognition elements) and thus selectivity for the receptor heterodimer. Most of the previous reports have shown compounds with only modest preference for heterodimers over monomers. In many cases, it has not been demonstrated that the two linked pharmacophores address two orthosteric-binding sites of two neighbouring protomers. GPCR crystal structures may leverage an effective development of novel molecular probes and drug candidates [48] , because they can be used for structure-based in silico docking screens, giving access to new chemotypes and, as a consequence, to new biological profiles. Furthermore, they can guide the evolution of novel ligands by providing insights into attractive and repulsive ligand–receptor interactions and the relative topology of crucial moieties. Both strategies can be performed based on either the crystal structure of a given GPCR or starting from a homology model of a structurally highly similar congener. Using the co-crystallized ligands eticlopride and NT(8-13) as fragments for the design of bivalent ligands, the recently resolved X-ray crystal structures of NTS 1 R, D 3 R and a β 1 -AR dimer combined with homology modelling enabled us to determine the relative disposition of the pharmacophores to each other and to identify suitable attachment points for the spacer units. The strategy allowed a rational, structure-guided development of bivalent D 2 R/NTS 1 R ligands. The compounds 1b - d , 2b - d and 3b - d show unprecedented selectivity (up to three orders of magnitude) and binding affinity in the picomolar range for cells coexpressing both GPCRs, compared with cells that only express D 2 Rs. Preparations of porcine striatal membranes were used to investigate the biological relevance of our bivalent ligands. Although differences between high- and low-affinity binding sites were smaller, biphasic-binding curves confirmed a bivalent-binding behaviour. A functional switch was observed for bivalent ligands containing a dopamine receptor agonist moiety. The compounds 3b and 3c behaved as agonists in cells singly expressing D 2 R inhibiting cAMP formation. However, no inhibitory effect on the NTS 1 R-promoted cAMP accumulation resulting from NTS 1 R activation by the NT(8-13) fragment was observed in D 2 R/NTS 1 R-coexpressing cells. Thus, the bivalent ligands 3b and 3c containing a D 2 R agonist pharmacophore behaved identical to bivalent ligands bearing a D 2 R antagonist moiety ( 2b and 2c ), pointing towards a NTS 1 R-dominated signalling behaviour within D 2 R/NTS 1 R heterodimers. Yet, the exact molecular mechanism underlying this phenomenon is not fully understood. In particular, the extremely high binding affinity could not be translated into activation potency. The observed cAMP accumulation may be caused by monovalent binding to NTS 1 R, if the bivalently bound D 2 R/NTS 1 R heterodimer is unable to activate G proteins. However, interpretation of the functional experiments is far from trivial, as the overall response results from the activation of mixed populations of D 2 R and NTS 1 R monomers, homomers and heteromers. Moreover when dealing with bivalent ligands, at least three different (and probably even more) binding modes have to be considered: a monovalent-binding mode to each protomer as well as a bivalent, receptor-bridging binding mode. As a second signalling pathway, we investigated the recruitment of β-arrestin-2. Employing an assay based on enzyme complementation, we could determine D 2 R-mediated β-arrestin-2 recruitment; while NTS 1 R-mediated engagement of β-arrestin-2 was only detectable in presence of the ProLink-tagged D 2 R. Compared with cells singly expressing D 2 Rs, coexpression and activation of NTS 1 R leads to a significant increase in potency. Thus, NTS 1 R protomer appears to dominate not only G protein coupling but also β-arrestin-2 recruitment in D 2 R/NTS 1 R-coexpressing cells. Importantly, bell-shaped dose–response curves were observed for the bivalent ligands 2b , c and 3b , c , whereas the structural analogues 2a and 3a with a shorter linker or a combination of two monovalent orthosteric ligands (quinpirole and NT(8-13)) showed regular sigmoid dose–response curves. In analogy to the binding behaviour of 2b , c and 3b , c (biphasic curves), the atypical dose–response relationship suggests a concentration-dependent contribution of different modes of receptor–ligand interactions. While it is not clear how exactly different binding modes influence the receptors’ capacity to recruit β-arrestin-2, the atypical dose–response curves obviously indicate that bivalent ligands with adequately designed spacer units display receptor activation characteristics distinct from monovalent ligands. Although the simultaneous presence of bivalent, receptor-bridging binding modes and monovalent-binding modes for bivalent ligands may represent a valid concept, we cannot exclude other, probably allosteric effects, leading to an altered binding and signalling behaviour. Even though the exact molecular mechanism underlying the atypical functional behaviour remains to be elucidated, our study demonstrates the successful development of bi-orthosteric bivalent ligands targeting D 2 R/NTS 1 R heterodimers with unique properties. Because our target receptors are of major relevance for the pathophysiology of neurological and psychiatric disorders including Parkinson’s disease and schizophrenia, the D 2 R/NTS 1 R heterodimer may be a promising pharmacological target [17] . The tissue selectivity of bivalent D 2 R/NTS 1 R ligands may confer high potency and reduced side effects. Presumably, the in vivo bioavailability of our compounds of types 1–3 will not be suitable for their use as a drug. However, our newly developed bivalent ligands represent powerful pharmacological tools and may serve as a starting point for the development of innovative imaging agents and drugs addressing GPCR heterodimers, as sophisticated drug-delivery systems are currently developed. Molecular modelling D 2 R/NTS 1 R dimer models were generated by superimposing both our recently described homology model of the D 2 R (ref. 40 ) (which was based on the D 3 R crystal structure [36] ) and the NTS 1 R crystal structure (PDB-ID 4BUO) [39] with the so far resolved crystal structures of GPCR dimers. For details on the selection process see Supplementary Note 1 and Supplementary Tables 1 and 2 . The final dimer model, created based on the crystal structure of the β 1 -AR dimer (PDB-ID 4GPO) [41] , was submitted to an energy minimization procedure as described previously [40] . Ligand positions were obtained in different ways. The coordinates of NT(8-13) in the crystal structure of NTS 1 R (ref. 39 ) were maintained for its position in the heterodimer model. The position of eticlopride was obtained by superimposing the crystal structure of D 3 R (ref. 36 ), including co-crystallized eticlopride, with our D 2 R homology model, followed by a transfer of the eticlopride coordinates to the D 2 R homology model. Coordinates of the remaining compounds were achieved by docking using AutoDock Vina [49] as described previously [40] . Out of the 20 best-ranked conformations, one final conformation for each ligand was selected based on the scoring function of AutoDock Vina, experimental data and a manual inspection followed by an additional energy minimization. The all-atom force field ff99SB (ref. 50 ) was used for receptors and NT(8-13) and the general AMBER force field (GAFF) [51] was used for the remaining ligands. A formal charge of +2 was assigned to NT(8-13), with the N-terminus and side chains of arginine protonated and the C-terminus deprotonated. A formal charge of +1 was assigned to the D 2 R ligands, here the basic nitrogen was protonated. Further details on heterodimer model generation, docking procedures and MD simulations are provided in Supplementary Notes 1–3; Supplementary Figs 1–4; and Supplementary Tables 1 and 2 . Snapshots of MD simulations are provided as Supplementary Data 1 , 2 , 3 . All figures were prepared using the UCSF Chimera package 1.10 (ref. 52 ). Synthesis and characterization of bivalent ligands Detailed schemes and conditions for the synthesis of the bivalent ligands 1a – d, 2a – f and 3a – f and the monovalent analogues 2g and 3g are provided in Supplementary Figs 16–18 . Detailed methods and characterization for all compounds and precursors are provided as Supplementary Methods . For nuclear magnetic resonance analysis of the small molecules described in this article, see Supplementary Figs 19–34 . Cell culture HEK 293 T cells (ATCC accession number CRL-11268) and HEK 293 cells stably expressing the EA-tagged β-arrestin-2 fusion protein (DiscoveRx) were maintained in DMEM/F-12 supplemented with 10% fetal bovine serum, 2 mM L -glutamine, 100 μg ml −1 penicillin, 100 μg ml −1 streptomycin and 150 μg ml −1 hygromycin for EA-β-arrestin-2 cells at 37 °C, 5% CO 2 (all cell culture reagents purchased from Invitrogen/Thermo Fisher Scientific). Cell lines were tested for mycoplasma contamination using the MycoAlert Plus detection kit (Lonza, Verviers, Belgium) on a regular basis. Receptor-binding experiments Receptor-binding studies were carried out in analogy to a previously described method [53] . Accordingly, competition-binding experiments with the human D 2L R were perfomed using preparations of membranes from HEK 293 T cells, which were transiently transfected with the D 2L R (from Missouri S&T cDNA Resource Center (UMR), Rolla, MO) using the Mirus TransIT-293 transfection reagent (purchased from MoBiTec, Goettingen, Germany). The assays were carried out in binding buffer (50 mM Tris pH 7.4, 5 mM MgCl 2 , 1 mM EDTA, 100 μg ml −1 bacitracin and 100 μg ml −1 soybean trypsin inhibitor) at a final volume of 200 μl with a protein concentration of 5–8 μg per assay tube, K D values of 0.048–0.060 nM and corresponding B max values of 960–970 fmol mg −1 , together with [ 3 H]spiperone (specific activity 81 Ci mmol −1 , PerkinElmer, Rodgau, Germany) at a final concentration of 0.20–0.25 nM. Binding experiments with the co-transfected receptors were performed using membrane preparations from HEK 293 T cells, which were transiently transfected (Mirus TransIT-293) with the D 2L R and NTS 1 R (from UMR) in the appropriate ratio of cDNA. Competition-binding experiments with the resulting homogenates of membranes coexpressing both receptors were carried out at a protein concentration of 1–8 μg per assay tube together with [ 3 H]spiperone at a final concentration of 0.10–0.25 nM. For the detailed investigation of the heterobivalent ligands membranes with receptor densities of D 2L R and NTS 1 R in the ratio of 1:2 ( K D values of 0.053–0.080 nM, B max =800 fmol mg −1 for D 2L R, 1,500–2,000 fmol mg −1 for NTS 1 R), 2:1 ( K D 0.040 nM, B max =2,000 fmol mg −1 D 2L R 1,000 fmol mg −1 NTS 1 R) and 3:1 ( K D 0.050 nM, B max =8,000 fmol mg −1 D 2L R, 2,500 fmol mg −1 NTS 1 R) were used. Competition-binding experiments with [ 3 H]neurotensin (final concentratrion 0.50 nM, specific activity 101 Ci mmol −1 ; PerkinElmer, Rodgau, Germany) were performed at a protein concentration of 2 μg per assay tube and relative expression levels of 2.5:1 ( B max =3,000 fmol mg −1 D 2L R, 1,200 fmol mg −1 NTS 1 R, K D 0.50 nM). Unspecific binding was determined in the presence of haloperidol (10 μM for D 2L R) or NT(8-13) (10 μM for NTS 1 R). Protein concentration was established by the method of Lowry using bovine serum albumin as standard [54] . Binding experiments with porcine striatal membranes were performed as described above together with [ 3 H]spiperone (final concentration 0.20–0.24 nM) at a protein concentration of 20 μg per tube (B max =220 fmol mg −1 D 2L R, 140 fmol mg −1 NTS 1 R, K D =0.090 nM). Data analysis The resulting competition curves of the receptor-binding experiments were analysed by nonlinear regression using the algorithms in PRISM 6.0 (GraphPad Software, San Diego, CA). For each individual experiment, the data were fitted using a monophasic competition model to provide an IC 50 value, which was then transformed into a K i value according to the equation of Cheng and Prusoff [55] . The monophasic fit was accepted, unless a biphasic competition model providing two individual values for K i high and K i low resulted in a statistically significant better fitting of the data (extra sum-of-squares F-test, P<0.05). cAMP BRET Assay HEK 293 T cells were transiently transfected with pcDNA3L-His-CAMYEL (ref. 43 ) (ATCC) and D 2S R and/or NTS 1 R at a cDNA ratio of 2:2 or 2:2:2 (unless indicated otherwise), respectively, using Mirus TransIT-293 transfection reagent. Resulting receptor expression levels were determined in saturation-binding experiments with membranes from transfected HEK 293 T cells and found to be 21±6 pmol mg −1 protein for D 2S R monoexpression, 25±13 pmol mg −1 for NTS 1 R monoexpression and 15±4 and 7.2±1.7 pmol mg −1 for D 2S R and NTS 1 R (1:1 transfection ratio) or 5.6±3.0 and 26±11 pmol mg −1 for D 2S R and NTS 1 R (0.5:3.5 transfection ratio), respectively in the coexpressing cells. 24 h post-transfection cells were seeded into white half-area 96-well plates at 2.0 × 10 4 cells per well and grown overnight. On the following day phenol red free medium was removed and replaced by PBS and cells were serum starved for 1 h before treatment. The assay was started by adding 10 μl coelenterazine-h (Promega, Mannheim, Germany) to each well to yield a final concentration of 5 μM. After 5 min incubation, compounds were added in PBS containing 50 μM forskolin (final concentration 10 μM). Reads of the plates started 15 min after agonist addition. BRET readings were collected using a CLARIOstar plate reader (BMG LabTech, Ortenberg, Germany). Emission signals from Renilla Luciferase and YFP were measured simultaneously using a BRET 1 filter set (475–30 nm/535–30 nm). BRET ratios (emission at 535–30 nm/emission at 475–30 nm) were calculated and dose–response curves were fitted by nonlinear regression using the algorithms of PRISM 6.0. Curves were normalized to basal BRET ratio obtained from dPBS (0%) and the effect of 10 μM forskolin (100%). β-Arrestin-2 recruitment assay The measurement of β-arrestin-2 recruitment stimulated by receptor activation was performed by utilizing the PathHunter assay purchased from DiscoveRx (Birmingham, UK) according to the manufacturer’s protocol. Accordingly, HEK 293 cells stably expressing the EA-tagged β-arrestin-2 fusion protein (provided by DiscoveRx) were transiently transfected with the ProLink(ARMS2-PK2)-tagged D 2S R (or the respective ARMS2-PK2-tagged D 2S R_D80A mutant) together with or without cotransfection of NTS 1 R at a cDNA ratio of 1:3 using Mirus TransIT-293 transfection reagent. Resulting receptor expression levels were determined in saturation-binding expriments with membranes from the same pool of cells and found to be 3.5±0.9 pmol mg −1 protein for D 2S R and 4.2±0.3 pmol mg −1 for NTS 1 R in the D 2 R/NTS 1 R coexpression and 3.5±1.2 and 11.5±3.3 pmol mg −1 for D 2S R_D80A and NTS 1 R, respectively for coexpression of the signalling incompetent D 2 R mutant together with NTS 1 R. 24 h after transfection, cells were detached using Versene (Invitrogen), 5,000 cells per well were seeded in 384-well plates and maintained at 37 °C, 5% CO 2 for 24 h. After incubation with different concentrations of test compounds (from 10 −15 to 10 −4 M final concentration) in duplicates for 5 h, the detection mix was added and incubation was continued for further 60 min. Chemiluminescence was determined with a CLARIOstar reader for microplates (BMG LabTech). Resulting responses were normalized to the maximum effect obtained with quinpirole (100%) and the basal response (vehicle, 0%), or relative to the response of NT(8-13) (100%) when the signalling incompetent D 2S R_D80A mutant was used. Dose–response curves were calculated by nonlinear regression using the algorithms of PRISM 6.0. Control experiments were performed using the same approach and transfection of ProLink(PK1)-tagged PAR 2 together with wild-type NTS 1 R. Under these conditions, NTS 1 R expression levels were determined to be 8.7±1.2 pmol mg −1 protein. Resulting responses were then normalized to the effect of the PAR 2 agonist f-LIGRLO-NH 2 . Data availability The data that support the findings of this study are available within the Supplementary Information files and/or from the corresponding authors upon request. How to cite this article: Hübner, H. et al . Structure-guided development of heterodimer-selective GPCR ligands. Nat. Commun. 7:12298 doi: 10.1038/ncomms12298 (2016).